Femtosecond electrons probing currents and atomic structure in nanomaterials The investigation of ultrafast electronic and structural dynamics in low-dimensional systems such as nanowires and two-dimensional materials requires femtosecond probes providing high spatial resolution and strong interaction with small volume samples. Low-energy electrons exhibit large scattering cross-sections and high sensitivity to electric fields, but their pronounced dispersion during propagation in vacuum so far prevented their use as femtosecond probe pulses in time-resolved experiments. Here, employing a laser-triggered point-like source of either divergent or collimated electron wave packets, we developed a hybrid approach for femtosecond point projection microscopy and femtosecond low-energy electron diffraction. We investigate ultrafast electric currents in nanowires with sub-100 femtosecond temporal and few 10 nm spatial resolutions, and demonstrate the potential of our approach for studying structural dynamics in crystalline single-layer materials. One- and two-dimensional (2D) crystalline materials have emerged as fundamental building blocks for nanoscale devices [1] , [2] , [3] . Compared with the respective bulk materials, the reduced dimensionality of the translational symmetry has profound effects on the ground state properties of nanomaterials as well as on the coupling between electronic, nuclear and spin degrees of freedom, dictating the dynamical behaviour. As all devices operate in states out of equilibrium, and as the dwell time of excited electrons in nanostructures is comparable to the time scale of typical relaxation processes, electron–lattice–spin interactions crucially determine the functionality of future nanodevices. A range of ultrafast laser-based techniques is nowadays available for probing the evolution of electronic, optical, structural and magnetic properties of solids after a sudden perturbation such as optical excitation, providing invaluable information on the mutual coupling of electronic, nuclear and spin degrees of freedom, as well as of transport properties. Despite femtosecond temporal resolution, the investigation of ultrafast processes in nanoscaled, low-dimensional systems additionally requires high spatial resolution [4] , [5] , [6] as well as high sensitivity sufficient for investigating small sample volumes, that is, femtosecond probe pulses strongly interacting with the sample. Electrons with sub-keV kinetic energies, here referred to as low-energy electrons, exhibit exceptionally high scattering cross-section and a de Broglie wavelength on the order of 1 Å, which, in principle, allows for achieving atomic resolution both in imaging as well as diffraction approaches. Whereas the spatial resolution of current techniques for time-resolved nanoscale imaging of electric fields relies on the near-field enhancement at nanostructures [5] , [6] , the high sensitivity of low-energy electrons to electric fields further permits the investigation of weak field distributions in the vicinity of nanoscale objects [7] . Although the generation of few-femtosecond electron pulses is readily achieved by photoemission [8] , [9] , [10] , [11] , the biggest challenge in using low-energy electrons as ultrafast probe is to maintain femtosecond duration of the electron pulses during delivery to the sample. Unlike optical laser pulses, femtosecond electron pulses suffer from temporal broadening in vacuum during propagation to the sample, especially at low energies [12] . Many-electron pulses can be strongly affected by space charge broadening due to Coulomb repulsion [13] . Furthermore, even single electron wave packets experience significant dispersive broadening depending on their initial energy distribution [14] . Temporal compression techniques can be used to obtain femtosecond many-electron pulses at a distant sample [15] , but have yet to be demonstrated for low electron energies. Alternatively, space charge broadening can be eliminated by using single electron pulses at high repetition rates [16] , [17] . Still, achieving femtosecond time resolution with dispersing sub-keV single electron pulses further requires considerable reduction of the propagation distances [18] , [19] . In the present study, we accomplish femtosecond time resolution by minimizing the electron propagation length down to the micrometre range in combination with using single electron pulses. We developed a compact hybrid approach for femtosecond low-energy electron diffraction (fsLEED) and femtosecond point projection microscopy (fsPPM) with electron energies in the range 20–1,000 eV. A laser-triggered metal nanotip provides a compact point-like source of coherent femtosecond electron wave packets [8] , [9] , [10] , [11] , optionally collimated for diffraction or spatially diverging for microscopy [7] , [19] , [20] . Employing the microscopy mode of operation, we investigate ultrafast currents in axially doped InP nanowires (NWs) with femtosecond temporal and nanometre spatial resolution. The potential of the diffraction mode to study ultrafast structural dynamics in 2D materials is demonstrated by recording high-quality diffraction images of single-layer graphene with femtosecond electron pulses. 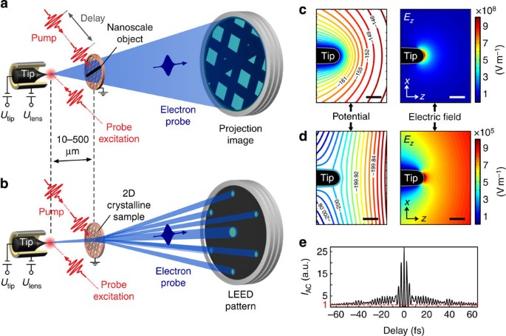Figure 1: Setup for time-resolved low-energy electron imaging and diffraction. Photoelectrons, generated from a nanotip by an ultrashort laser pulse, are accelerated towards the sample positioned several micrometres away from the tip for either (a) point projection microscopy of nanoscale object (divergent electron beam), or (b) low-energy electron diffraction of 2D crystalline samples (collimated beam). A pump laser pulse, variably delayed from the electron probe, photoexcites the sample for time-resolved experiments. An electrostatic lens is used to switch from the divergent imaging mode (c, curved potential lines and strong inhomogeneous fieldEz) to the collimated diffraction mode (d, flattened potential and reduced electric fieldEz), each at a tip voltageUtip=−200 V, but different lens voltagesUlens,im=−200 V andUlens,dif=−730 V, respectively. The scale bars indicate 100 nm. Temporally confined electron emission is verified by measuring the interferometric autocorrelation photocurrentIACfrom the tip, revealing a third-order emission process (e). Experimental concept Figure 1a,b show the two operation modes for fsPPM and fsLEED, respectively. A tungsten nanotip is positioned at sub-millimetre distances in front of the sample. Photoelectrons are generated by focusing an ultrashort laser pulse on the negatively biased tip and are accelerated towards the grounded sample. For time-resolved pump–probe experiments, a second laser pulse is focused on the sample under 45° and the arrival time between the two pulses can be varied with an optical delay stage. Projection images and diffraction patterns are recorded with a microchannel plate (MCP) as electron detector positioned 10 cm behind the sample (more details on the setup are described in the Methods section). Figure 1: Setup for time-resolved low-energy electron imaging and diffraction. Photoelectrons, generated from a nanotip by an ultrashort laser pulse, are accelerated towards the sample positioned several micrometres away from the tip for either ( a ) point projection microscopy of nanoscale object (divergent electron beam), or ( b ) low-energy electron diffraction of 2D crystalline samples (collimated beam). A pump laser pulse, variably delayed from the electron probe, photoexcites the sample for time-resolved experiments. An electrostatic lens is used to switch from the divergent imaging mode ( c , curved potential lines and strong inhomogeneous field E z ) to the collimated diffraction mode ( d , flattened potential and reduced electric field E z ), each at a tip voltage U tip =−200 V, but different lens voltages U lens,im =−200 V and U lens,dif =−730 V, respectively. The scale bars indicate 100 nm. Temporally confined electron emission is verified by measuring the interferometric autocorrelation photocurrent I AC from the tip, revealing a third-order emission process ( e ). Full size image For collimation and energy tuning, we place the tip inside an electrostatic microlens, being either directly coated onto the shaft of the tip [21] or using a metal-coated ceramic microtube. Examples of the potential and electric field E z in the vicinity of the tip’s apex for the imaging and diffraction mode are plotted in Fig. 1c,d , respectively. The electric field strength at the apex can be adjusted via the lens voltage independent of the tip voltage, enabling energy tuning at a constant emission current [21] . For diffraction, the electron beam is collimated by flattening the potential field lines around the apex. This is accompanied by a reduction of DC field enhancement, and no field emission is possible in the diffraction mode. However, the nanotip still enhances the optical laser field, leading to localized photoemission from the apex [22] . The photoemission process at the tip is characterized by measuring an interferometric autocorrelation of the photocurrent with the tip as nonlinear medium [23] , as plotted in Fig. 1e . The peak/baseline ratio of 27:1 reveals a third-order emission process, implying that the electron emission is temporally confined to ~3 fs in case the tip is illuminated with 5-fs laser pulses (see Methods). Femtosecond point projection microscopy We performed fsPPM measurements on axially doped p - i - n InP NWs [24] with a 60-nm-long i -segment in the centre, spanning across 2 μm holes in a gold substrate, see Fig. 2a . A projection image of a single NW recorded in field emission mode at a distance d =20 μm and at 90 eV electron energy is shown in Fig. 2b . Noticeably, the wire diameter appears bright and much larger than its projected real space diameter. Owing to the low electron energies, the projection image is in fact not a shadow image of the spatial shape of the nanoscale object, but is rather revealing the local electrostatic field in the object's near-surface region deflecting the electron trajectories [7] , [25] . These static lensing effects critically depend on extrinsic parameters such as the tip field [7] , [26] and intrinsic parameters such as work function variations, for example, between the NW and the substrate. 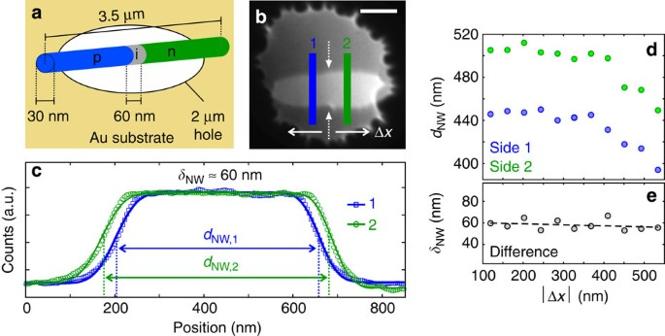Figure 2: Point projection microscopy of axially doped NWs. InP NWs (radius 15 nm, length 3.5 μm) withp-i-naxial doping profile and 60 nmi-segment in the centre are spanned across 2 μm holes in a gold substrate (a). Instead of being a real shadow image of the objects shape, projection images are strongly influenced by local fields surrounding the NW, which becomes apparent by the bright NW projection recorded in constant current (field emission) mode at a tip voltage of −90 V (b; scale bar: 500 nm). In addition, a spatial inhomogeneity of the projected diameter along the NW with a step ofδNW≈60 nm from the left to the right side of the NW centre (marked by the white arrows inb) is observed (c). The projected diameter is plotted indas a function of distance from the NW centre for both left side (blue) and right side (green) of the NW, illustrating the lensing effects occurring when approaching the edges of the hole. The diameter differenceδNWbetween the left and right side of the NW, as plotted ine, remains constant at a value ofδNW≈60 nm. This corresponds to a potential difference in the 100 meV range and a difference in the radial field around the NW on the order of a few MV m−1, as found by simulations (see Methods). Figure 2: Point projection microscopy of axially doped NWs. InP NWs (radius 15 nm, length 3.5 μm) with p - i - n axial doping profile and 60 nm i -segment in the centre are spanned across 2 μm holes in a gold substrate ( a ). Instead of being a real shadow image of the objects shape, projection images are strongly influenced by local fields surrounding the NW, which becomes apparent by the bright NW projection recorded in constant current (field emission) mode at a tip voltage of −90 V ( b ; scale bar: 500 nm). In addition, a spatial inhomogeneity of the projected diameter along the NW with a step of δ NW ≈60 nm from the left to the right side of the NW centre (marked by the white arrows in b ) is observed ( c ). The projected diameter is plotted in d as a function of distance from the NW centre for both left side (blue) and right side (green) of the NW, illustrating the lensing effects occurring when approaching the edges of the hole. The diameter difference δ NW between the left and right side of the NW, as plotted in e , remains constant at a value of δ NW ≈60 nm. This corresponds to a potential difference in the 100 meV range and a difference in the radial field around the NW on the order of a few MV m −1 , as found by simulations (see Methods). Full size image Furthermore, we observe a step of the projected NW diameter d NW close to the NW centre. Figure 2c shows line profiles through the NW at two different positions along the wire, revealing a difference of d NW,1 − d NW,2 ≈60 nm in the projected sample plane. This contrast can be explained by different electric fields surrounding the NW induced by spatial variations of the work function. Although the step is due to the change in the materials properties at the p – i – n junction, the superimposed gradual increase of the projected NW width is due to lensing effects at the edges of the hole in the substrate. The DC projection image of the p – i – n NW in Fig. 2b is analysed by taking line profiles at different positions along the NW and fitting a double error function to the data. The projected NW diameter increases from the substrate contacts at the hole edges towards the NW centre (indicated by the white dashed line in Fig. 2b , as plotted in Fig. 2d ) and saturates close to the centre where the i -segment is expected. Noticeably, we observe a constant difference in the projected width between both sides of the NW, δ NM (Δ x )= d NW,1 (Δ x )− d NW,2 (Δ x ), at every distance Δ x from the NW centre of δ NM (Δ x )=60 nm, see Fig. 2e . This inhomogeneity clearly indicates different surface fields on both sides of the NW, as expected for different doping types. By performing numerical simulations of the electron trajectories taking into account all experimental parameters, we can reproduce the recorded projections and relate the observed NW diameters to specific distributions of the potential and electric field at the sample (see Methods). We find that the experimentally observed step corresponds to a difference of the local potential in the 100 meV range. Owing to the nanometre dimensions, such small potential differences result in electric fields on the order of several MV m −1 . As the trajectories of low-energy electrons are highly sensitive to such field strength, point projection microscopy provides a sensitive technique for the investigation of electrostatic fields of nanoscale systems. In case of semiconducting NWs with constant radii, the homogeneity of their projected width depends on the specific surface condition, that is, the doping level, crystal structure and chemical composition [27] , [28] , [29] . Employing femtosecond low-energy electron wave packets in an optical pump–electron probe scheme, we map the transient change of the NW diameter Δ d NW after fs laser excitation. 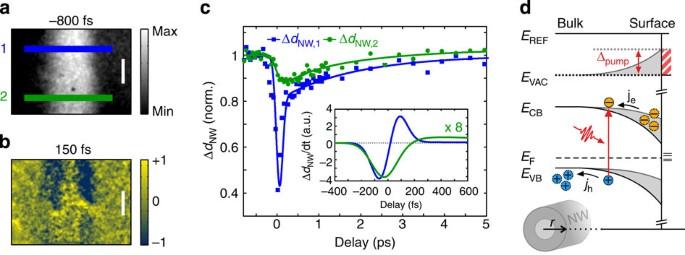Figure 3: Femtosecond imaging of ultrafast photocurrents in InP NWs. (a) Projection image of the same NW as inFig. 2b) recorded in pulsed fsPPM mode at negative time delays. Photoecxitation by an ultrashort laser pulse leads to a transient, spatially inhomogeneous change of the projected NW diameter (b, normalized difference plot). (Data recorded at 70 eV electron energy; scale bars: 500 nm). Different dynamical behaviour and amplitudes of the transient diameter change ΔdNWare observed for thep- andn-doped segments along the NW (c), where an empirical three-exponential function was fitted to the data. Both segments show a fast initial photo-induced effect with 10–90 rise times in thep- andn-segments of 140 and 230 fs, respectively, followed by multi-exponential decay on the fs-to-few picosecond time scale. As ΔdNWis directly proportional to the transient electric field change, the derivate ΔdNW/dtplotted in the inset incis a direct measure of the instantaneous photocurrent inside the NW. Surface states cause effective radial doping leading to band bending at the NW surface as sketched ind, where r is the radial coordinate, causing a radial photocurrent of electrons,je, and holes,jh, after photoexcitation. This leads to a pump-induced transient shift Δpumpof the conduction band edgeECBand valence band edgeEVB, and hence a shift of the vacuum levelEvac(red shaded area), compared to the reference levelEref(given by the environment), with the magnitude of the shift depending on the specific band bending and doping level. Figure 3a shows the fsPPM image of the same NW as in Fig. 2b , 800 fs before optical excitation. At temporal overlap, we observe a clear pump-induced, spatially inhomogeneous change of d NW , which axially varies along the NW, as apparent in the difference image taken at 150 fs in Fig. 3b . The dynamics of the photo-induced change of the projected NW diameter in both segments are plotted in Fig. 3c . We observe a difference in the maximum amplitudes of the transient signal of for the two segments. Both transients have a fast initial rise, followed by a multi-exponential decay on the femtosecond to picosecond time scale. Figure 3: Femtosecond imaging of ultrafast photocurrents in InP NWs. ( a ) Projection image of the same NW as in Fig. 2b ) recorded in pulsed fsPPM mode at negative time delays. Photoecxitation by an ultrashort laser pulse leads to a transient, spatially inhomogeneous change of the projected NW diameter ( b , normalized difference plot). (Data recorded at 70 eV electron energy; scale bars: 500 nm). Different dynamical behaviour and amplitudes of the transient diameter change Δ d NW are observed for the p - and n -doped segments along the NW ( c ), where an empirical three-exponential function was fitted to the data. Both segments show a fast initial photo-induced effect with 10–90 rise times in the p - and n -segments of 140 and 230 fs, respectively, followed by multi-exponential decay on the fs-to-few picosecond time scale. As Δ d NW is directly proportional to the transient electric field change, the derivate Δ d NW / dt plotted in the inset in c is a direct measure of the instantaneous photocurrent inside the NW. Surface states cause effective radial doping leading to band bending at the NW surface as sketched in d , where r is the radial coordinate, causing a radial photocurrent of electrons, j e , and holes, j h , after photoexcitation. This leads to a pump-induced transient shift Δ pump of the conduction band edge E CB and valence band edge E VB , and hence a shift of the vacuum level E vac (red shaded area), compared to the reference level E ref (given by the environment), with the magnitude of the shift depending on the specific band bending and doping level. Full size image In addition to the intentional axial doping, we expect the NWs to exhibit an effective radial doping induced by surface states, pinning the Fermi level and leading to band bending far into the NW [28] , as sketched in Fig. 3d . The associated surface space charge field strongly differs for the different doping types, being larger for the p - than for the n -doped segment [28] . In particular, the effective radial doping profile of the p -segment changes from p -doping in the NW bulk to n -doping at the NW surface, whereas the n -segment exhibits a radial n - n + profile, leading to an effective n - n + doping axially along the NW surface, which reduces the axial doping contrast without photoexcitation. After above-band-gap photoexcitation, electrons and holes homogeneously generated in the NW bulk are radially separated by the surface field, leading to radial photocurrents j e and j h , respectively. This carrier separation, however, transiently reduces the surface band bending due to screening of the space charge fields [30] , leading to a transient shift of the vacuum level, indicated by the red shaded area in Fig. 3d . As this is accompanied by a change Δ E NW of the local electric field at the NW surface, we can monitor these shifts by a transient change of the projected NW diameter being directly proportional to Δ E NW (see Supplementary Fig. 1 ). Consequently, the derivative Δ d NW /d t shown in the inset of Fig. 3c is a direct measure of the photo-induced radial currents inside the NW. The spatial inhomogeneity and the different dynamics of the photo-induced effect result from the local doping contrast along the NW. The relaxation of the photo-induced effect is governed by the transport properties and the electronic structure of the NW segments. A detailed discussion of the different relaxation processes is beyond the scope of this letter. Here we limit the discussion to the fast initial dynamics, which provide an upper limit for the time resolution of our fsPPM setup. Considering that the built-in radial electric field is on the order of several 10 kV cm −1 for heavily doped wires [28] , we assume a drift velocity of the photoexcited carriers as high as the saturation velocity in InP, which is 7 × 10 6 cm s −1 (ref. 31 ). With a wire radius of 15 nm, we expect a drift time of ~200 fs, which agrees well with the observed 10–90 rise times of 140 fs and 230 fs of p - and n -segment, respectively. Hence, we interpret the fast initial dynamics as direct measure of radial photocurrent in the NW and conclude that the observed dynamics reflect the carrier dynamics and is not limited by the temporal resolution of our instrument, which according to simulations is expected to be <50 fs in the imaging mode [14] . These results demonstrate the feasibility of fsPPM as a novel approach for probing ultrafast currents on the nanoscale with fs temporal resolution. Femtosecond LEED We further want to discuss the suitability of our setup to study ultrafast structural dynamics in low-dimensional materials by fsLEED. Very recently, Gulde et al. [18] demonstrated the capability of low-energy electrons to study the structural dynamics of a bilayer system on the ps time scale. Here we introduce an alternative approach for the implementation of time-resolved LEED using the potential of our electron gun design to realize very short propagation distances of the focused beam on micrometre-length scales, therefore minimizing temporal broadening of the electron pulse. The capability of our setup to record high-quality LEED patterns of monolayer samples is shown by focusing the electron beam onto single-layer graphene suspended over a lacey carbon film (Ted Pella, Inc.). 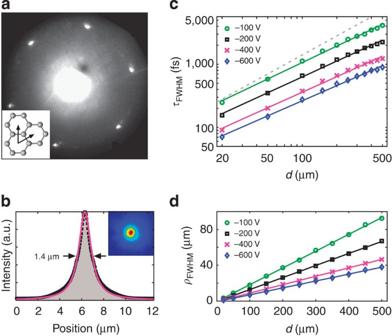Figure 4: LEED of free-standing monolayer graphene with fs electron pulses. LEED pattern of monolayer suspended graphene recorded in transmission at a tip–sample distance of 500 μm and 650 eV electron energy (a, inset: hexagonal lattice of graphene). Owing to the confined emission area and small propagation distances, the pulsed electron beam can be collimated down to a spot size of 1-2 μm (FWHM) on the sample (b), shown here ford=200 μm. The electron pulse durationτFWHMincis obtained by the FWHM of the arrival time distribution of single electron wave packets for distancesdbetween 20 and 500 μm, and electron energies from 100 to 600 eV. A sub-linear dependenceτFWHM∝dγwithγ≈0.83 is observed (γ≈1 for the dashed line). Equivalently, the dependence of the electron spot sizeρFWHM, defined as the FWHM of the radial position distribution at the sample position, is plotted ind, which is in good agreement with the experimental observations. The dependence on the tip voltage results from the underlying focusing conditions. Figure 4a shows a diffraction pattern recorded in transmission at d= 500 μm and 650 eV electron energy exhibiting the six-fold symmetry of the 2D hexagonal lattice of graphene [32] . It is noteworthy that even for monolayer samples, diffraction patterns of very high quality can be recorded at very low electron dose rate (<1 electron Å −2 s −1 ) owing to the high scattering cross-section of sub-keV electrons [33] . Hence, the implementation of fsLEED for studying structural dynamics in single- and few-layer systems is clearly favourable compared with conventional high-energy femtosecond electron diffraction [34] . Figure 4: LEED of free-standing monolayer graphene with fs electron pulses. LEED pattern of monolayer suspended graphene recorded in transmission at a tip–sample distance of 500 μm and 650 eV electron energy ( a , inset: hexagonal lattice of graphene). Owing to the confined emission area and small propagation distances, the pulsed electron beam can be collimated down to a spot size of 1-2 μm (FWHM) on the sample ( b ), shown here for d =200 μm. The electron pulse duration τ FWHM in c is obtained by the FWHM of the arrival time distribution of single electron wave packets for distances d between 20 and 500 μm, and electron energies from 100 to 600 eV. A sub-linear dependence τ FWHM ∝ d γ with γ ≈0.83 is observed ( γ ≈1 for the dashed line). Equivalently, the dependence of the electron spot size ρ FWHM , defined as the FWHM of the radial position distribution at the sample position, is plotted in d , which is in good agreement with the experimental observations. The dependence on the tip voltage results from the underlying focusing conditions. Full size image To study the structural dynamics of such 2D materials after photoexcitation with an ultrashort laser pulse, electron pulses with a length significantly below 1 ps at the sample position are desirable in the diffraction mode. We investigate the electron wave packet propagation in fsLEED mode by numerical simulations for various tip–sample distances and electron energies (see Methods). The key properties of the electron wave packet, namely its temporal profile and its transverse coherence length, critically depend on the field distribution around the tip axis. As those change with tip–sample distance and with the tip and lens voltages, we define an experimentally meaningful focusing condition to compare the results obtained for the electron pulse duration and spot size at the sample. From the experimental point of view, it is reasonable to assume a constant resolution in the diffraction patterns, implying a constant transverse coherence length l t . In Fig. 4c , the expected full width at half maximum (FWHM) electron pulse duration τ FWHM is plotted as a function of tip–sample distance for different electron energies, where the focusing condition is adjusted to provide a l t of ~30 nm (described in more detail in the Methods section). The pulse duration decreases sub-linearly with shorter propagation length, τ FWHM ∝ d γ , with γ ≈0.83, which can be explained by the distance-dependent reduced inhomogeneity of the acceleration field at the apex in the diffraction mode [14] . So far, the shortest possible distances in the diffraction mode are ~150 μm, restricted by vacuum breakthrough at the electron lens, limiting the electron pulse duration to ~300 fs, see Fig. 4c . Future improvements of the lens design should allow distances as close as 20 μm, that is, distances comparable to the imaging mode, pushing the time resolution of diffraction experiments to the 100 fs range. We also calculate the electron spot size at the sample and compare it with the experiment. Owing to the absence of space charge and due to the confined emission area, the electron pulses can be focused down to a few micrometres on the sample, as shown in Fig. 4b , where we plot the radially averaged profile revealing a spot size ρ FWHM of 1.4 μm of the collimated electron beam. The calculated FWHM spot size, plotted in Fig. 4d , linearly decreases with the tip–sample distance down to a few micrometres, where the slope α =Δ ρ FWHM /Δ d , that is, the beam divergence, depends on the tip voltage according to α ∝ ( U tip ) −1/2 (see Methods), reflecting our assumption of constant coherence in the diffraction pattern. Small deviations between simulation and measurement can be due to differences in the probability distributions used for the emission statistics and due to slightly different focusing conditions. Ultimately, such small electron spot sizes avoid spatial averaging over large domains with multiple crystal orientations, providing an ultrafast structural probe with single-crystal selectivity on micrometre-length scales. We realized a novel approach for fsPPM and fsLEED using low-energy electron pulses photo-generated from a metal nanotip. We demonstrated the excellent capability of fsPPM for nanoscale imaging of small electric fields around semiconductor NWs with femtosecond time resolution. In general, fsPPM enables direct spatiotemporal probing of ultrafast processes on nanometre dimensions in the near-surface region of nanostructures, such as ultrafast carrier dynamics and currents, dynamics of interfacial fields, as well as ultrafast plasmonics. Ultimately, taking advantage of the high sensitivity of sub-keV femtosecond electron pulses combined with the magnification provided by PPM, our approach potentially allows the investigation of ultrafast phenomena on length scales down to the molecular level [35] . In addition to real space imaging, low-energy electron pulses are ideal probes for studying structural dynamics of 2D crystalline materials on the femtosecond time scale by time-resolved diffraction. Using a nanotip as miniaturized electron gun for fsLEED allows to reduce the electron propagation length to the 100-μm range and to minimize temporal broadening to the 100-fs range. Combining the high surface sensitivity of low-energy electrons with femtosecond time resolution, fsLEED will reveal real-time information on structural dynamics and energy transfer processes in monolayer 2D materials and inorganic [36] as well as organic [37] composite heterostructures thereof. Experimental setup A detailed sketch of the setup is depicted in Fig. 5 . Depending on the specific application, two different laser systems are employed: an ultra-broadband 800 nm Ti:Sa oscillator operating at 80 MHz repetition rate, providing 5 fs pulses with ~2 nJ pulse energy, and a cavity-dumped 800 nm Ti:Sa oscillator with variable repetition rate up to 2 MHz delivering 16 fs pulses with 30 nJ pulse energy. For generation of photoelectrons from the tip, a part of the laser output is focused on the tip to a 3- to 4-μm spot size (1/ e 2 radius), with the polarization along the tip axis. For time-resolved pump–probe measurements, the second output part is focused onto the sample under an angle of 45°. The arrival time between the electron probe and the optical pump pulse is varied by an optical delay stage integrated in the pump arm. The interferometric autocorrelation in Fig. 1e was measured at 80 MHz repetition rate with 5 fs pulses and a fluence of 0.14 mJ cm −2 , with the collimated electron beam at 400 eV electron energy and a copper grid as anode at a distance of ~1 mm. The fsPPM data were measured at 1 MHz repetition rate with 16 fs pulses, with a fluence of 0.7 mJ cm −2 focused on the tip and 0.2 mJ cm −2 to pump the NWs. An integration time of 2 s was used for each projection image and the data are averaged over ten subsequent scans for every delay point. Temporal overlap in Fig 3a–c is defined by the empirical multi-exponential fit to the data. For the diffraction data, 5 fs pulses at 80 MHz repetition rate were focused on the tip at a fluence of 0.22 mJ cm −2 , and diffraction patterns are recorded with an integration time of 0.5 s and averaged over 100 frames. 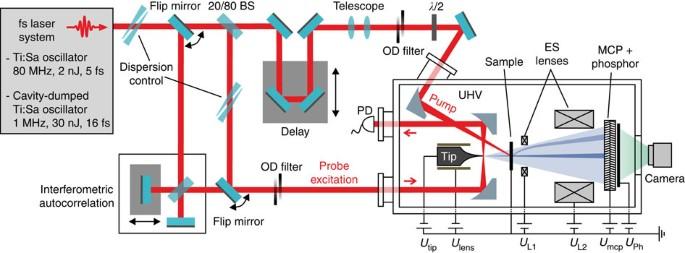Figure 5: Schematic of the experimental setup. The setup for fsPPM and fsLEED is shown. Figure 5: Schematic of the experimental setup. The setup for fsPPM and fsLEED is shown. Full size image Nanotips with 20–100 nm radii are electrochemically etched from 150 μm polycrystalline tungsten wire. The outer surface of a ceramic tube with an inner (outer) diameter of 200 μm (500 μm) was coated with 100 nm chromium as electron lens. The tip is centred inside the tube and protrudes ~150 μm from the lens. Bias voltages U tip and U lens up to −2 kV are applied to the tip and the electrostatic microlens depending on the operation mode. Photoelectrons are accelerated towards the grounded sample and amplified by a MCP detector ( U mcp ) combined with a phosphor screen ( U Ph ). Two additional electrostatic lenses at positive bias voltages U L1 and U L2 are installed behind the sample to collimate the large diffraction angles obtained in LEED on the plane MCP screen. In the imaging mode, these lenses are switched off. A scientific camera is used to record the images outside ultrahigh vacuum. A piezo-driven ten-axis positioning system is used for precise alignment of the electron gun and sample inside the laser focuses, and relative to each other. All experiments are performed under ultrahigh vacuum conditions (10 −10 mbar). Numerical simulations The numerical simulations of the point projection images as well as the electron pulse duration and spot size at the sample in the fsLEED mode were performed with a similar approach as described in ref. 14 . A finite element method is used to model the electrostatic field between the electron gun and the sample, and, in the case of PPM, the detector. Propagation of single electron wave packets inside the electrostatic field is simulated classically using a Runge–Kutta algorithm. The shape of the tip apex is modelled by a half sphere with a 15-nm radius and the shaft has an half-opening angle of 13.5°. To simulate projection images, we calculate the classical single electron trajectories in three dimensions with cartesian coordinates x ={ x , y , z }, see Fig. 6 , with the NW spanning across a round hole in x direction and the tip pointing along the z direction. Hence, we choose the x - z plane as symmetry plane to reduce the computational cost. The sample is modelled by a 200-nm thin metal layer with a 2-μm hole centred on the z axis. The NW is formed by a cylinder with radius r NW embedded in the sample. We compute the electron trajectories for a regular grid of emission angles θ x and θ y in x and y direction, respectively, assuming electron emission normal to the tip surface. A single electron energy is considered, as a finite energy distribution has an insignificant effect on the spatial resolution in the projection images compared with other experimental effects such as mechanical vibrations and drifts during image acquisition. Projection images are generated by analysing the arrival positions of all trajectories on the detector plane. Assuming equal emission probability for all trajectories, the image intensity is calculated by phase space mapping between the initial condition and the detector arrival position, integrated over the regular grid of initial conditions. 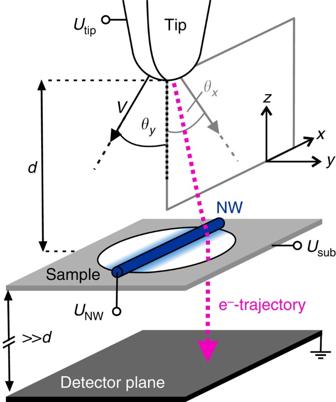Figure 6: PPM simulation geometry. Electrons with initial velocityvand emission anglesθxandθyinxandydirection, respectively, are accelerated to the sample, and possibly deflected by electric fields in the sample vicinity. Projection images are then evaluated in the distant detector plane. Figure 6: PPM simulation geometry. Electrons with initial velocity v and emission angles θ x and θ y in x and y direction, respectively, are accelerated to the sample, and possibly deflected by electric fields in the sample vicinity. Projection images are then evaluated in the distant detector plane. Full size image To account for work function variations between the NW and the substrate as well as to the environment (for example, due to different materials), bias voltages U sub and U NW,0 are applied to the sample substrate and the NW, respectively. In addition, a potential distribution accounting for axial work function variations along the NW, for example, due to doping effects, can be applied to the NW. To simulate an axial p - i - n doping structure, we model the potential distribution of the NW along the x direction by with the (cumulative) probability function the respective potentials and of the p - and n -doped segments, and with x 0 and D x being the position and width of the i -segment along the x direction, respectively. The potential distribution U NW and corresponding electric fields E x and E y are exemplified in Supplementary Fig. 2 . The resulting effect on the projection images recorded in the detector plane is illustrated in Supplementary Fig. 1 for two different potential distributions. The simulation of electron pulse duration and spot size in the fsLEED operation mode follow the procedure described in ref. 14 , assuming cylindrical symmetry and additionally including the electron lens. For the weak-field regime in the case of multi-photon photoemission, we can neglect the effect of the optical laser field on the propagation. We choose Gaussian distributions for the electron kinetic energy E , for the emission angle θ 1 (emission normal to the tip surface), as well as for the momentum distributions at each emission point within and outside the simulation plane, implemented by the angles θ 2 and θ 3 , respectively, see Fig. 7 . In particular, the out-of-plane angel θ 3 can be mapped onto the velocity of the electron by v ′= v ·cos ( θ 3 ), effectively reducing the initial electron energy, as the out-of-plane momentum does not affect the arrival time but only induces a precession of the trajectories and their arrival positions around the z axis (no fields in azimuthal direction due to cylindrical symmetry). In the present study, the simulations are calculated for a mean energy E 0 =0.5 eV and s.d. σ E =0.25 eV, σ θ 1 =10° and σ θ 2 = σ θ 3 =30° (angles all distributed around zero), adopting the distributions given in ref. 38 . 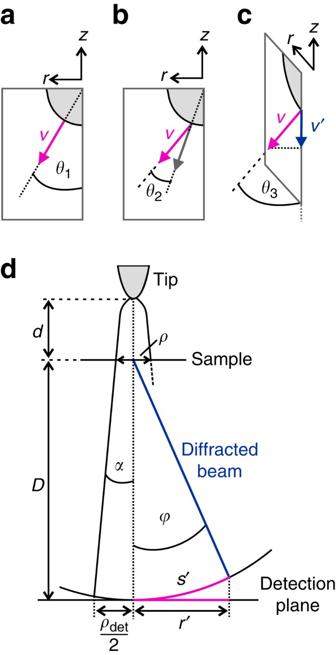Figure 7: Simulation geometry for LEED. Definition of emission anglesθ1(a), normal to the tip surface, andθ2(b) andθ3(c) accounting for the in- and out-of-plane momentum distributions, respectively. (d) Sketch of the geometric parameters used to define the focusing condition. Figure 7: Simulation geometry for LEED. Definition of emission angles θ 1 ( a ), normal to the tip surface, and θ 2 ( b ) and θ 3 ( c ) accounting for the in- and out-of-plane momentum distributions, respectively. ( d ) Sketch of the geometric parameters used to define the focusing condition. Full size image In diffraction experiments, the transverse coherence length is usually defined as the ratio between the width of the diffraction spot on the detector, ρ det , and its radial position r ′, where a is the lattice constant of the investigated sample [34] . For a spherical detector, r ′ can be defined as the projection of the arc length s ′ on a planar detection plane, see Fig. 7 , and is proportional to the diffraction angle ϕ , that is, r ′ ∝ sin ( ϕ ) in first approximation. According to Bragg’s law and the momentum energy relation for non-relativistic electrons with kinetic energy eU tip , we then obtain r ′ ∝ ( U tip ) −1/2 . Hence, a constant coherence length for all electron energies requires r ′ ∝ ( U tip ) −1/2 and likewise ρ ∝ ( U tip ) −1/2 for the spot size at the sample in the case of field-free propagation between sample and detector. In the simulations, this focusing condition is realized by calculating the required electric field strength at the apex, which leads to the desired target spot sizes. The calculations shown in Fig. 4b,d are computed assuming an initial spot size with a s.d. of σ ρ =15 μm at U tip =−100 V and d =200 μm. The beam divergence α given by the slopes in Fig. 4d show the desired dependence α ∝ ( U tip ) −1/2 as plotted in Supplementary Fig. 3 . We thus obtain a corresponding spot size on the detector of ρ det =0.37 mm at a distance of 10 cm. With the Bragg angle of ϕ =29.7°, giving r ′=0.057 mm, and using the lattice constant a =2.465 Å of graphene, we obtain a transverse coherence length of l t ≈38 nm for the above given values. In the same way, we obtain a coherence length of l t ≈35 nm at U tip =−600 V (with σ ρ =6.12 μm). fsPPM data analysis For each delay frame, the projected width of the NW d NW was fitted with a double error function and averaged over line scans, separately in the blue and green regions indicated in Fig. 3a . The dynamics of the extracted values as a function of the delay time τ plotted in Fig. 3c ) were best fitted empirically with three exponentials convolved with a Gaussian. Here, Θ (t) is the Heaviside function, A n and γ n are the amplitudes and decay rates of the different decay contributions, respectively, and τ 0 is the zero time delay. The constant offsets A 0 and A ∞ represent the initial value (before pump) and long-lived contribution to d NW ( τ ), respectively. Samples InP NWs with axial p - i - n doping structure are grown as described in ref. 24 and mechanically transferred to a gold substrate with a regular pattern of 2 μm holes. Single-layer graphene electron microscopy support films are purchased from Ted Pella, Inc. (product number 21710) and used without any subsequent treatment. How to cite this article: Müller, M. et al. Femtosecond electrons probing currents and atomic structure in nanomaterials. Nat. Commun. 5:5292 doi: 10.1038/ncomms6292 (2014).